Postmortem examination of patient H.M.’s brain based on histological sectioning and digital 3D reconstruction Modern scientific knowledge of how memory functions are organized in the human brain originated from the case of Henry G. Molaison (H.M.), an epileptic patient whose amnesia ensued unexpectedly following a bilateral surgical ablation of medial temporal lobe structures, including the hippocampus. The neuroanatomical extent of the 1953 operation could not be assessed definitively during H.M.’s life. Here we describe the results of a procedure designed to reconstruct a microscopic anatomical model of the whole brain and conduct detailed 3D measurements in the medial temporal lobe region. This approach, combined with cellular-level imaging of stained histological slices, demonstrates a significant amount of residual hippocampal tissue with distinctive cytoarchitecture. Our study also reveals diffuse pathology in the deep white matter and a small, circumscribed lesion in the left orbitofrontal cortex. The findings constitute new evidence that may help elucidate the consequences of H.M.’s operation in the context of the brain’s overall pathology. Henry G. Molaison, known in the medical literature as Patient H.M., began experiencing minor epileptic seizures when he was 10 years old and major seizures when he was 15. The underlying aetiology of his seizure disorder remains uncertain; a minor head injury earlier in his childhood may have been a contributing factor. The worsening seizures not only compromised his health but also disrupted his school performance and social life; as a young adult, epilepsy affected his ability to work and function independently. In 1953, because even very high doses of available anticonvulsant medications were ineffective, the 27-year-old underwent a neurosurgical procedure performed by William Beecher Scoville, with the intention of decreasing the impact of his seizures on his quality of life. Following the surgery, in which portions of the medial temporal lobes (MTL) were resected bilaterally, H.M.’s seizure frequency was reduced, although he remained on anticonvulsant medication. There was, however, an unexpected and profound effect on his behaviour: after recovering from the operation, he was unable to recollect routine events during his hospital stay and did not recognize the staff that attended him assiduously. In spite of this obvious impairment, H.M.’s intellectual abilities and personality appeared to be unaffected [1] . His language and perceptual skills were intact; moreover, based on tests done 10 months after the operation, when the seizures had subsided, his IQ was above average [2] . His attentional and working memory capacities were normal, and he was able to hold items in mind by actively rehearsing them. He could not, however, consolidate and store this information in long-term memory. For example, he was able to carry on a conversation proficiently but several minutes later would be unable to remember having had the exchange or the person with whom he spoke. Further testing gradually revealed some forms of preserved learning and memory. Notably, he demonstrated intact motor skill learning [3] , [4] , classical conditioning [5] , perceptual learning [6] , and visuoperceptual priming [7] , although he was oblivious to the fact that he had repeatedly performed these tasks with the experimenter and had no declarative knowledge of the learning experience [8] , [9] , [10] . H.M. demonstrated this new procedural learning through performance but could not verbalize what he had learned. Researchers concluded that this nondeclarative learning relied on memory circuits separate from those in the MTL region and that it did not require conscious memory processes [10] . H.M.’s semantic memory for the years preceding the operation was preserved, but he could not retrieve any episodic, autobiographical memories from that time. Instead, he conceptualized his memories of friends and experiences, relating only general knowledge about people and places [6] , [11] , [12] , [13] . Postoperatively, H.M. was profoundly impaired in learning new episodic and semantic information, but gradually over time he acquired a few new facts and snippets of knowledge about celebrities, likely due to repeated exposure to this information [14] , [15] . The defining deficit in H.M.’s case was an inability to form new declarative memories, a syndrome that became indelibly linked to the bilateral resection of the hippocampus and neighbouring MTL structures [16] . H.M. made his debut into the medical literature as a case described in a seminal publication, which is one of the most cited articles in the medical literature [1] . His case acquired broad significance in the field largely because the neurological substrate of memory was unknown at the time of his operation and H.M. provided the first conclusive evidence for the involvement of the hippocampal complex. Scoville’s intraoperative impressions, however, were the only estimate of the extent of H.M.’s lesions. Before H.M.’s surgery, Scoville published several illustrations of his surgical technique [16] , [17] ; these sketches showed how metal retractors were inserted through two trephine holes ∼ 1 inch above the orbits to lift the frontal lobes. Postoperative drawings reflected Scoville’s intent to carry out a symmetrical medial resection reaching as far as 8 cm from the midpoints of the tips of the temporal lobes [1] , [18] . This procedure would have removed the uncus, amygdala and the hippocampal complex, including the parahippocampal gyrus (based on the drawings, the ablation affected the anterior calcarine cortex, which contains the representation for the peripheral visual field) [1] . At the time of the operation it was not possible to evaluate postsurgical outcomes with neuroimaging; thus, Scoville’s drawings were only speculative. The first modern CT scans of H.M.’s brain published in 1984 did not clearly reveal the nature and extent of tissue damage in the temporal lobes [2] ; however, a better view of H.M.’s brain was obtained in 1992 and 1993 using magnetic resonance imaging (MRI) [19] . MRI scans revealed that the lesion was symmetrical as Scoville had planned, but was less extensive than his estimate [19] . It included the medial temporal polar cortex, most of the amygdaloid complex and entorhinal cortex (EC), and about half of the rostro-caudal extent of the intraventricular segment of the hippocampal formation (dentate gyrus, hippocampus and subiculum). Portions of the ventral perirhinal cortex were spared, and the parahippocampal cortex appeared largely intact. The frontal, parietal and occipital cortices had a generally normal appearance, and neocortical atrophy was slight and consistent with H.M.’s age. The authors pointed out that any residual hippocampal tissue had been significantly deafferented by the removal of the EC and was, therefore, unlikely to have preserved function. A higher-resolution series of MRI scans conducted when H.M. was in his mid-seventies revealed a number of age-related morphological changes: cortical thinning, atrophy of deep grey matter structures and a large volume of abnormal white matter (WM) and deep grey matter [20] . Most of these alterations appeared to be of recent origin, and were attributed to acquired medical conditions, including hypertension. The MRI scans collected in vivo lacked sufficient resolution to reveal the exact anatomical boundaries of the MTL lesions, and to characterize secondary changes. H.M. died of respiratory failure on 2 December 2008. Direct examination of the brain, combined with postmortem imaging [21] , [22] , represented the opportunity to address the limitations of previous non-invasive MRI studies [19] , [20] and to provide a clear anatomical verification of the lesion and the pathologic state of surrounding areas. Our goal was to create a detailed three-dimensional (3D) model of the whole brain from high-resolution anatomical images so that we could revisit, by virtual dissection, Scoville’s surgical procedure and localize the anatomical borders of the lesion in the temporal lobe. The data also supported accurate measurements of H.M.’s remaining hippocampus and assessment of the tissue at the microscopic level. Because it was critical to preserve an organized archive of images and histological slices to conduct retrospective studies, we designed the protocols and instrumentation necessary to collect and image a complete series of histological sections through the whole brain. Detailed mapping at the microscopic level and 3D measurements within the digital model of the brain showed that H.M. had retained a significant portion of the hippocampus that appears histologically intact in both hemispheres. Dissection and tomographic imaging of the brain specimen The ventral aspect of the brain, after the removal of the leptomeninges, clearly showed the scars of the operation on both hemispheres ( Fig. 1 ). On the surface, the right and left lesions appeared roughly symmetrical in length and in respect to anatomical landmarks; however, the full extent of the injury could only be determined upon dissection. Serial sectioning and direct tomographic imaging was performed in the coronal plane in alignment with the anterior and posterior commissures (AC-PC); these interhemispheric fibre bundles run perpendicular to the major axis of the brain and form the reference points for a widely-used standard radiologic stereotaxic system [23] . AC-PC alignment ensured that histological sections could be compared with previous scans of H.M.’s brain [19] , [20] , those of other patients [24] , [25] , [26] , [27] , and neuroimaging data from population-based studies [28] . Rigorous stereotaxic orientation also guaranteed that any interhemispheric differences in the length of the lesion or in the morphology of the spared hippocampus noted in the histological images reflected actual anatomical asymmetry rather than unconventional planes of section. 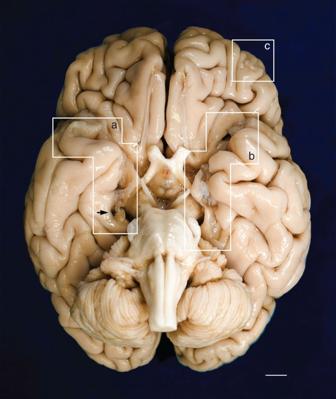Figure 1: Ventral surface of H.M.’s brain. The fixed specimen was photographed after removal of the leptomeninges. Evidence of the surgical lesions in the temporal lobes is highlighted by white geometric contours (a, b). A mark produced by the oxidation of one of the surgical clips inserted by Scoville is visible on the parahippocampal gyrus of the right hemisphere (black arrow). (c) encloses a lesion in the orbitofrontal gyrus that affects the cortex and WM. Marked cerebellar atrophy is consistent with H.M.’s long-term treatment with phenytoin. Scale bar, 1 cm. Figure 1: Ventral surface of H.M.’s brain. The fixed specimen was photographed after removal of the leptomeninges. Evidence of the surgical lesions in the temporal lobes is highlighted by white geometric contours (a, b). A mark produced by the oxidation of one of the surgical clips inserted by Scoville is visible on the parahippocampal gyrus of the right hemisphere (black arrow). (c) encloses a lesion in the orbitofrontal gyrus that affects the cortex and WM. Marked cerebellar atrophy is consistent with H.M.’s long-term treatment with phenytoin. Scale bar, 1 cm. Full size image The results of our examination are based on 2,401 digital anatomical images and selected corresponding histological sections that were collected at an interval of 70 μm over the course of an uninterrupted 53-hour procedure. The series of digital images of the block’s surface was obtained using a digital camera mounted directly above the microtome stage. Volumetric reconstruction from these images was the basis for subsequent visualization and 3D measurements along arbitrary planes. The dissection of the brain was video-recorded and streamed live on the web to permit scientific scrutiny and to foster public engagement in the study [29] . 3D anatomical measurements in the MTL Using the 3D measurement tools in AMIRA (FEI Visualization Science Group, Burlington, MA, USA) we calculated the distance in each hemisphere from the anterior tip of the temporal lobe to the posterior boundary of the surgical lesion on each side. This limit was marked by the most anterior coronal anatomical images that did not show any sign of disruption in the normal anatomy, which was confirmed in corresponding stained histological slices. The lesion followed a straight, but slightly oblique path relative to the long axis of each hemisphere; measured along this axis, its length was 54.5 mm and 44.0 mm in the left and right hemispheres, respectively. The value for the left hemisphere was consistent with earlier measurements made on H.M.’s MRI scans acquired in 1992–1993 (ref. 19 ) and 2002–2004 (ref. 20 ). The lesion in the right hemisphere as measured in our postmortem data was 7 mm shorter than in the above-mentioned reports that were based on in vivo imaging. The borders of the surgical resection were clearly demarcated in the anatomical and histological images; the latter clearly showed that the WM underlying the excised medial temporal cortex was also damaged ( Fig. 2 ). We identified a small portion of the superior-most region of the EC in both hemispheres based on its distinctive cytoarchitecture; specifically, 0.03 cm 3 and 0.11 cm 3 for the left and right hemispheres, respectively (these values correspond approximately to 1.7% and 6.5% of the normal volume, based on published MRI estimates [30] ). Portions of the centromedial nucleus of the amygdala were also preserved ( Fig. 2h,i ). 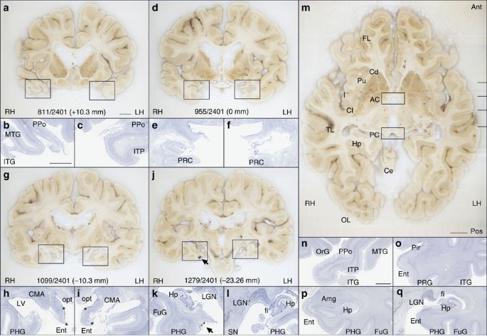Figure 2: Anatomical and histological views of the lesion and residual hippocampus. (a,d,g,j) Cross-sectional anatomy of patient H.M.’s MTL shown at four different levels. The values below the tissue indicate the section number and in parenthesis, the distance from the origin of the standard coordinate system23(positive if the level is anterior to the anterior commissure, negative if posterior). Scale bar, 1 cm. (b,c), (e,f), (h,i), (k,l): close-up images acquired from thionin-stained tissue slices; these panels illustrate histological detail for the selection boxes ina,d,g,j, respectively. Scale bar, 5 mm. (m) Horizontal cross-sectional view reconstructed orthogonally from the original coronal images showing the correct alignment of the anterior and posterior commissures. (n–q): normal anatomy and histology of the MTL at the levels shown for the brain of patient H.M. The images were derived from brain slices belonging to a neurologically normal, age-matched individual. Scale bar, 5 mm. PPo, planum polare; MTG, middle temporal gyrus; ITG, inferior temporal gyrus; ITP, inferior temporopolar cortex; PRC, perirhinal cortex; CMA, centromedial amygdala; opt, optic tract; LV, lateral ventricle; PHG, parahippocampal gyrus; Ent, entorhinal cortex; LGN, lateral geniculate nucleus; Hp, hippocampus; FuG, fusiform gyrus; fi, fimbria; SN, substantia nigra; FL, frontal lobe; Cd, caudate; Pu, putamen; I, insula; AC, anterior commissure; Cl, claustrum; TL, temporal lobe; PC, posterior commissure; Ce, cerebellum; OL, occipital lobe; OrG, orbital gyrus; Pir, pirifom cortex; Amg, amygdala. The asterisks delimit the entorhinal cortex. Figure 2: Anatomical and histological views of the lesion and residual hippocampus. ( a , d , g , j ) Cross-sectional anatomy of patient H.M.’s MTL shown at four different levels. The values below the tissue indicate the section number and in parenthesis, the distance from the origin of the standard coordinate system [23] (positive if the level is anterior to the anterior commissure, negative if posterior). Scale bar, 1 cm. ( b , c ), ( e , f ), ( h , i ), ( k , l ): close-up images acquired from thionin-stained tissue slices; these panels illustrate histological detail for the selection boxes in a , d , g , j , respectively. Scale bar, 5 mm. ( m ) Horizontal cross-sectional view reconstructed orthogonally from the original coronal images showing the correct alignment of the anterior and posterior commissures. ( n – q ): normal anatomy and histology of the MTL at the levels shown for the brain of patient H.M. The images were derived from brain slices belonging to a neurologically normal, age-matched individual. Scale bar, 5 mm. PPo, planum polare; MTG, middle temporal gyrus; ITG, inferior temporal gyrus; ITP, inferior temporopolar cortex; PRC, perirhinal cortex; CMA, centromedial amygdala; opt, optic tract; LV, lateral ventricle; PHG, parahippocampal gyrus; Ent, entorhinal cortex; LGN, lateral geniculate nucleus; Hp, hippocampus; FuG, fusiform gyrus; fi, fimbria; SN, substantia nigra; FL, frontal lobe; Cd, caudate; Pu, putamen; I, insula; AC, anterior commissure; Cl, claustrum; TL, temporal lobe; PC, posterior commissure; Ce, cerebellum; OL, occipital lobe; OrG, orbital gyrus; Pir, pirifom cortex; Amg, amygdala. The asterisks delimit the entorhinal cortex. Full size image The extent of the spared hippocampus measured along the horizontal axis of the brain (which in our study coincided with the AC–PC line) was 23.6 mm in the left hemisphere and 24.3 mm in the right. Our measurements included the alveus and the thin band of WM that encapsulates the posterior end of the hippocampus; the fimbria was excluded from our delineations. The discrepancy between these new values and those obtained from earlier MRI data (19 and 22 mm, respectively) is small and can be explained by differences in the quality of the image data [19] . These linear measurements, however, do not fully account for the geometry of H.M.’s spared hippocampus. The high-resolution anatomical volume that we created from microtome images allowed us to inspect the MTL from multiple angles, revealing that the posterior hippocampus was bent steeply in the dorso-medial direction ( Fig. 3 ). This curvature is a normal feature of the periventricular portion of the hippocampus in the human brain, while the most anterior portion, which is immediately posterior to the amygdala and adjacent to the EC, is aligned to the horizontal plane (or major axis) of the hemisphere. 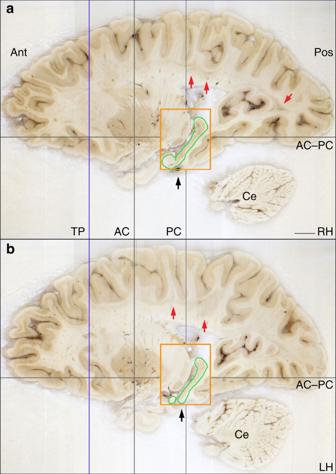Figure 3: Sagittal views of the right (a) and left (b) hemispheres reconstructed from the original series of coronal microtome images. The grey lines intersect at the origin of the origins of the standard coordinate system23used for the orientation of the specimen. The blue line indicates the most anterior level of the temporal lobes (the temporal poles, which are damaged are not shown in this image). The orange rectangle represents the bounding box that contains the posterior spared hippocampus (outlined in green), the widest extent of which is at a more medial level than this image shows. The black arrows identify the level at which a surgical clip was positioned on a blood vessel. The red arrows indicate the presence of lesions in the subcortical WM. AC, plane of the anterior commissure; PC, plane of the posterior commissure; AC–PC, ideal plane at the level of both the AC and PC; Ce, cerebellum; LG, lateral geniculate nucleus; Pu, putamen; TP, temporal pole; RH, right hemisphere; LH, left hemisphere. Scale bar, 1 cm. Figure 3: Sagittal views of the right (a) and left (b) hemispheres reconstructed from the original series of coronal microtome images. The grey lines intersect at the origin of the origins of the standard coordinate system [23] used for the orientation of the specimen. The blue line indicates the most anterior level of the temporal lobes (the temporal poles, which are damaged are not shown in this image). The orange rectangle represents the bounding box that contains the posterior spared hippocampus (outlined in green), the widest extent of which is at a more medial level than this image shows. The black arrows identify the level at which a surgical clip was positioned on a blood vessel. The red arrows indicate the presence of lesions in the subcortical WM. AC, plane of the anterior commissure; PC, plane of the posterior commissure; AC–PC, ideal plane at the level of both the AC and PC; Ce, cerebellum; LG, lateral geniculate nucleus; Pu, putamen; TP, temporal pole; RH, right hemisphere; LH, left hemisphere. Scale bar, 1 cm. Full size image Measuring the dorso-ventral oblique length of the posterior segment of H.M.’s hippocampus rather than along the AC–PC line produced higher values, specifically, 36.0 mm for the left hemisphere and 40.0 mm for the right. The values were greater when our calculations took curvature into account: in this case, the actual ‘geodesic’ length of the preserved hippocampus amounted to 45.4 mm in the left hemisphere and 47.2 mm in the right ( Fig. 4 ). 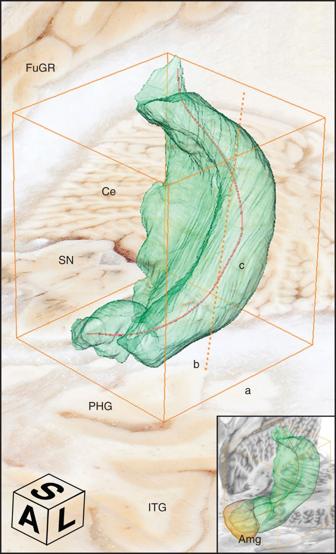Figure 4: Triangulated 3D surface reconstruction of H.M.’s spared left hippocampus. The orange bounding box delimits the dimensions of the structure; different segments indicate different measurements; a: anterior-to-posterior extent in the coronal plane, b (dotted): major diagonal axis, c: anatomical length. The compass cube (A: anterior, L: lateral, S: superior) also functions as scale bar: 5 mm. The insert at the bottom right shows a similarly constructed model from the brain of a neurologically normal subject (78-year-old female donor; volume of the right hippocampus=3.04 mm3; total brain weight 1,278). Ce, cerebellum; FuGR, fusiform gyrus of right hemisphere; IT, inferior temporal gyrus; SN, substantia nigra; Amg, amygdala. Figure 4: Triangulated 3D surface reconstruction of H.M.’s spared left hippocampus. The orange bounding box delimits the dimensions of the structure; different segments indicate different measurements; a: anterior-to-posterior extent in the coronal plane, b (dotted): major diagonal axis, c: anatomical length. The compass cube (A: anterior, L: lateral, S: superior) also functions as scale bar: 5 mm. The insert at the bottom right shows a similarly constructed model from the brain of a neurologically normal subject (78-year-old female donor; volume of the right hippocampus=3.04 mm 3 ; total brain weight 1,278). Ce, cerebellum; FuGR, fusiform gyrus of right hemisphere; IT, inferior temporal gyrus; SN, substantia nigra; Amg, amygdala. Full size image The fact that multiple results can be obtained based on different measuring criteria makes it necessary to establish a clear terminology to describe the anatomy of H.M.’s lesion and the remaining hippocampus in relation to previous reports. In the context of this communication, we refer to the extent of H.M.’s hippocampus and related structures as their linear span in the rostro-caudal direction. This measure can be obtained simply by multiplying the number of tomographic images by the interval between them (that is, slice thickness). The anatomical length of the hippocampus is different and depends on its 3D shape and orientation in the brain. With this distinction in mind, our findings can be more easily reconciled with previous reports that were based on low-resolution scans, where only the extent of the hippocampus was actually measured [19] . The level of sampling and image quality afforded by the current study represents a significant advance over the first clinical MRI that was performed with H.M. [19] . At that time, the two-dimensional (2D) MRI sequences produced 4–5-mm thick slabs with a 1-mm gap between each slice and an in-plane resolution slightly better than 1 mm per voxel; a T1-weighted 3D MRI scan was also acquired and produced non-isotropic voxels (1 × 1 × 3.2 mm). In these early scans, the boundaries of the posterior hippocampus were blurred by partial volume effects (the presence of multiple tissue types or structures in single large MRI voxels). In a more recent MRI study with H.M., Salat et al. [20] calculated the volume of tissue ascribed to the posterior hippocampus (voxel size: 1 mm × 1 mm × 1.3 mm) and obtained values of 0.65 cm 3 for the left hemisphere and 0.88 cm 3 for the right. We repeated these measurements based on manual delineations made on three orthogonal views of the digital anatomical reconstruction, and determined that 2.02 cm 3 of hippocampal tissue (including the cornu ammonis, the dentate gyrus and the subiculum) was spared in the left hemisphere and 1.96 cm 3 in the right. The comparison should be interpreted with caution in view of the fact that sufficient normative data on hippocampal volume based on our new postmortem methodology is not yet available. The labelled fields representing the posterior hippocampus in each hemisphere were used to compute triangulated surface models for visualization and shape analyses ( Fig. 4 ). Histology Regularly spaced tissue sections through the brain were selected at an interval of 1.26 mm; these were mounted on large-format glass slides (5 × 7 in) and stained using thionin. Nissl staining with thionin showed preservation of neuronal cell bodies in CA1, CA2, CA3, CA4 and the subiculum of the hippocampal formation, posterior to the surgical lesion ( Fig. 5 ). 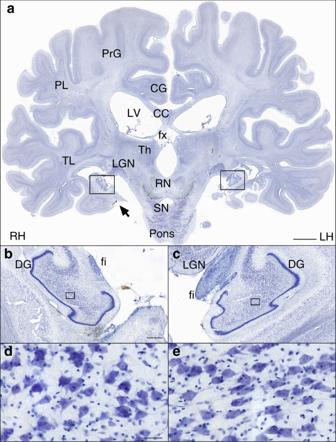Figure 5: Thionin-stained histological section at the level of the lateral geniculate nuclei. (a) Whole section. Scale bar, 1 cm. (b,c) Higher-magnification cross-sectional image of the dentate gyrus of the spared hippocampus. The fimbria is visible below the lateral geniculate nucleus. Scale bar, 1 mm. (d,e) × 20 magnification image of neurons in the CA4 region of the hippocampus (in the location of the box). Scale bar, 50 μm. PrG, precentral gyrus; PL, parietal lobe; CG, cingulate gyrus; LV, lateral ventricle; cc, corpus callosum; fx, fornix; Th, thalamus; TL, temporal lobe; LG, lateral geniculate nucleus; RN, red nucleus; SN, substantia nigra; DG, dentate gyrus; fi, fimbria. Figure 5: Thionin-stained histological section at the level of the lateral geniculate nuclei. ( a ) Whole section. Scale bar, 1 cm. ( b , c ) Higher-magnification cross-sectional image of the dentate gyrus of the spared hippocampus. The fimbria is visible below the lateral geniculate nucleus. Scale bar, 1 mm. ( d , e ) × 20 magnification image of neurons in the CA4 region of the hippocampus (in the location of the box). Scale bar, 50 μm. PrG, precentral gyrus; PL, parietal lobe; CG, cingulate gyrus; LV, lateral ventricle; cc, corpus callosum; fx, fornix; Th, thalamus; TL, temporal lobe; LG, lateral geniculate nucleus; RN, red nucleus; SN, substantia nigra; DG, dentate gyrus; fi, fimbria. Full size image Given that H.M. required surgery because of epilepsy and that there was partial response to the surgical intervention, it is of interest that the typical neuropathologic hallmarks associated with idiopathic temporal lobe epilepsy (granule cell dispersion in the dentate gyrus, neuronal loss from the pyramidal cell layer particularly in area CA4) were not present in the residual hippocampus. Pathologic anatomy beyond the MTL While the general size and cortical folding of the cerebral hemispheres appeared normal for an individual of H.M.’s age, multiple WM lesions consistent with lacunar infarctions were present. Cerebellar atrophy was also evident, likely a consequence of long-term exposure to Dilantin (phenytoin sodium), which was part of H.M.’s seizure management pre- and postoperatively [31] , [32] . Review of the MRI scans and histological sections demonstrated a spectrum of additional lesions in the WM ( Fig. 6 ). We also discovered a small focal lesion in the left lateral orbital gyrus, which was visible on the surface ( Fig. 1 c) and involved both cortex and underlying WM ( Fig. 7 ). 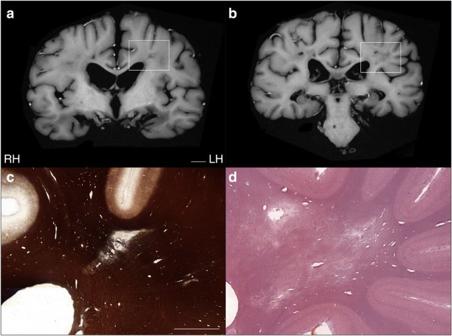Figure 6: Deep WM pathology. (a,b) Lesions in the deep WM were visible in postmortem T1-weighted MRI images acquiredex situ(scale bar, 1 cm) and were confirmed by myelin silver-impregnation40,46(c) and haematoxylin and eosin (H&E) staining (d). Scale bar, 5 mm. Figure 6: Deep WM pathology. ( a , b ) Lesions in the deep WM were visible in postmortem T1-weighted MRI images acquired ex situ (scale bar, 1 cm) and were confirmed by myelin silver-impregnation [40] , [46] ( c ) and haematoxylin and eosin (H&E) staining ( d ). Scale bar, 5 mm. 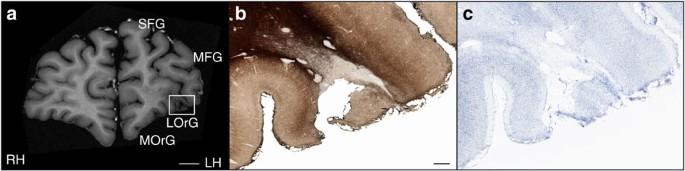Figure 7: Lesion in the left frontal lobe. The reconstructed anatomical volume revealed a small lesion in the lateral orbital gyrus of the left frontal lobe. This is the only lesion affecting the gross structure of the cerebral cortex outside of the MTL. (a) T1-weighted MRI of the fixed brain acquiredex situbefore cryo-sectioning. Scale bar, 1 cm. The same lesion is shown in histological material that was stained for myelinated fibres40,46(b) and neuronal cell bodies (c). Scale bar, 1 mm. Full size image Figure 7: Lesion in the left frontal lobe. The reconstructed anatomical volume revealed a small lesion in the lateral orbital gyrus of the left frontal lobe. This is the only lesion affecting the gross structure of the cerebral cortex outside of the MTL. ( a ) T1-weighted MRI of the fixed brain acquired ex situ before cryo-sectioning. Scale bar, 1 cm. The same lesion is shown in histological material that was stained for myelinated fibres [40] , [46] ( b ) and neuronal cell bodies ( c ). Scale bar, 1 mm. Full size image The 3D microscopic model of H.M.’s brain contained clues that help understand the surgery performed in 1953. Scoville approached the MTL of both hemispheres through two small trephine holes ( ∼ 3.8 cm in diameter) drilled above the orbits [17] . The ablation of the tip of the temporal lobe, the uncus and the amygdala was made with a scalpel; the sharp edge of the resections is noticeable in the anatomical and histological images ( Fig. 2d–f ). The more posterior MTL tissue was removed by suction; the fact that the periventricular portion of the hippocampus escaped the ablation can be explained by tracing the trajectory of the suction tube. Based on the reconstructed volume, it is clear that Scoville reached beyond and below the posterior hippocampus as indicated by the position of the surgical clip in the sagittal view of each hemisphere ( Fig. 3 ), although the placement of the clips was also contingent on the pattern of the surface vasculature. We could reliably identify only a very minimal amount of EC in H.M.’s brain based on cytoarchitecture. The EC (via its superficial layers) is the gateway to the hippocampus for the inflow of information from the cerebral cortex and subcortical nuclei. The hippocampus has reciprocal connections to neocortical areas that deliver the original input via the deep layers of the EC and parahippocampal gyrus, creating a loop that supports the consolidation of long-term memories. Our study confirmed that this circuit was severely compromised by the ablation. The hippocampus and EC also connect directly (that is, monosynaptically) to specific brain regions such as the nucleus accumbens, amygdala, cingulate cortex and orbitofrontal cortex. Input to and from the hippocampus is arranged along its anatomical length (as defined in this communication) according to an anterior-to-posterior functional gradient. For example, the amygdala is connected to anterior sections of the EC and hippocampus, while the visual cortex (largely residing in the occipital, parietal, lateral and ventral temporal lobes) is functionally linked to the posterior hippocampus. This organization is also reflected in the topography of differential gene expression and specific functional activation [33] , [34] , [35] . According to these maps, and based on the gradient of connectivity within the MTL and with other brain structures, the hippocampus appears broadly subdivided into an anterior segment that supports emotion, stress and sensorimotor integration, and a posterior part dedicated to declarative memory and neocortex-supported cognition [36] , [37] . According to this model, the almost complete removal of the EC in both hemispheres, resulting in severe disconnection of the remaining hippocampus, would have made a more significant contribution to H.M.’s declarative memory impairment than the ablation of the anterior hippocampus. The excision of the anterior hippocampus, together with the bulk of the amygdala, may explain H.M.’s dampened expression of emotions, poor motivation and lack of initiative [19] . The fact that he was impaired in reporting internal states such as pain, hunger and thirst and his apparent lack of initiative was ascribed to the almost complete removal of the amygdala, although it remains difficult to distinguish between direct injury to the amygdala and disruption of connections into and out of this complex structure [6] , [38] . The sparing of the posterior segment of the parahippocampal cortex may validate observations of H.M.’s preserved visual perception, perceptual learning and perceptual priming [6] , [39] . A detailed architectonic survey of occipital, parietal and ventral temporal areas [40] , [41] could provide new clues about the neural circuits H.M. engaged during the performance of numerous perceptual tasks. Histological staining revealed neuronal integrity in the CA4 field of the remaining hippocampus [42] and a normal compact pattern of the granule cell layer of the dentate gyrus ( Fig. 5 ). These findings raise interesting questions regarding the functional viability of H.M.’s remaining hippocampal tissue because according to established models of hippocampal connectivity, the gap in the MTL created by the surgery would have interrupted crucial connections to and from the posterior hippocampus. Additional quantitative analyses involving unbiased stereological methods can provide information regarding neuronal size and number [43] in this region. Combined with molecular approaches such as antibody staining to assess synaptic density, patterns of gliosis, and the integrity of afferent and efferent fibres, these studies could contribute further insight on the intrinsic and long-range connectivity of the human hippocampus. The lesion on the left frontal lobe was circumscribed to a small area within the left lateral orbital gyrus ( Fig. 1 c), and it involved the cortical ribbon as well as the underlying WM ( Fig. 7 ). Because of the removal of all leptomeninges as part of the preparation of the brain prior to sectioning, it is not possible to determine the status of the immediate subpial zone in the area of the lesion, which would have assisted in discriminating a mechanical laceration from a vascular injury. As mentioned above, Scoville performed the removal of deep MTL structures while each frontal lobe was retracted to provide access to the deeper temporal structures; thus, judging from the orientation of the ablation with respect to the position of the trephine holes, the scar in the left prefrontal cortex could plausibly have been created at the time of the surgery. In the course of the initial fixation, when the specimen was suspended upside down, the damaged portion of the temporal lobes collapsed; this geometrical artefact of fixation, combined with the relative shrinkage of the whole specimen during histological processing, should be considered when our resultsare compared with previous MRI scans obtained in vivo . It should be noted, however, that fixation, combined with cryoprotection, produced only an estimated 5–7% reduction in volume of the whole brain and these gross changes did not affect the morphology of the spared hippocampus. Attempts to provide structure–function correlations based on the postmortem evaluation of H.M.’s MTL require a parallel assessment of age-related neuropathologic processes that developed progressively in his brain. MRI demonstrated extensive WM T2-hyperintensities, which were not related to the surgery; these were confirmed in histological sections ( Fig. 6 ). Although H.M. suffered a minor head injury before age 10, this kind of event does not typically produce long-lasting traumatic injuries that can be subsequently detected radiologically, especially in the absence of clinical signs. Rather, the nature and distribution of observed WM pathology suggest the manifestation of microvascular disease associated with hypertension. Diagnostic neuropathologic evaluation is still required to determine the types and burden of abnormalities and disease processes that occurred independently of the surgery as a result of aging and related to other aetiologies. The purity and severity of H.M.’s memory impairment, combined with his willingness to participate in testing, made his case study uniquely influential in the field of memory research, as reflected in the broad range of scientific publications built on the studies to which he contributed [19] . During life, H.M. was the best-known and possibly the most studied patient in modern neuroscience; the availability of a large and organized collection of slices and digital anatomical images through the whole brain provides an unprecedented opportunity for collaborative and retrospective studies to continue [22] , [44] . The archive of images will also constitute a permanent digital trace for the case that defined two generations of memory research and that will likely remain as emblematic for neuroscience in the future as it is today. Ethics statement The study was reviewed and approved by one of UC San Diego’s Institutional Review Boards in accordance with the requirements of the Code of Federal Regulations for the Protections of Human Subjects. The removal and preservation of H.M.’s brain at autopsy, as well as disclosure of protected health information about him, was authorized by his legally appointed representative. Preparation of the brain Shortly after his death, H.M’s body was transported to the Anthinoula A. Martinos Center for Biological Imaging, in Charlestown, MA, where 9 h of in situ scanning was performed [21] . Following this imaging session, an autopsy was conducted; the brain removed, weighed (the total brain weight was 1,300 g) and then fixed in standard buffered formalin (4% formaldehyde; postmortem interval of ∼ 14 h). The brain was fixed for 10 weeks at 4 °C with three changes of fixative during that time; it was suspended upside down, hung by the basilar artery. When the tissue was firm enough, the brain was immersed in fixative laying on a cushion of hydrophilic cotton. Subsequently, multiple series of MRI scans of the fixed specimen were acquired in 3T and 7T scanners [21] . H.M.’s brain was transported to The Brain Observatory in February 2009, where fixation in formaldehyde continued for 2 more months. After this additional period of fixation, the brain was imaged in a 1.5 T General Electric (GE) Excite MRI scanner using an eight-channel transmit-receive head coil ( Figs 6a,b and 7a ). We used a T1-weighted, 3-D Inversion-Recovery Fast Gradient Echo (IR-FSPRG) sequence (image matrix: 512 × 512; Slice thickness: 1mm; FOV: 256; TE: 15; 18 excitations, or NEX. Duration of the scan: ∼ 7 hours). During the scan the brain was soaked in formaldehyde solution and contained in a watertight Plexigas chamber designed to fit inside the coil above mentioned. Following MRI, the brain was immersed in solutions of increasing concentration of sucrose; specifically, 10, 20 and 30% in 4% formaldehyde solution, phosphate-buffered to pH 7.4. Treatment with sucrose lasted ∼ 10 months: it was meant to minimize the formation of ice crystals and reduced the risk of creating cracks when the brain was frozen. Following fixation and cryoprotection, the leptomeninges were removed and the brain was embedded in a rectangular cast of 10% gelatin. The whole-brain-gelatin block was chilled to −40 °C by immersion in recirculating isopentane (2-methylbutane) using a custom-built insulated chamber. As the brain froze, the temperature of the solvent was constantly monitored and recorded via a probe connected to a personal computer running a custom programme (Labview, National Instruments Inc. Austin, TX, USA). The brain was thoroughly frozen after ∼ 5 h, when the temperature of the block and that of the surrounding fluid reached a stable equilibrium, based on probe data. The frozen block was firmly attached to the stage of a heavy-duty sliding microtome (Polycut SM 2500; Leica Microsystems Inc., Buffalo Grove, IL) and kept frozen by an assembly of interlocking hollow cuffs that transferred heat through a continuous flow of cold ethanol; the alcohol was recirculated and maintained at −40 °C by a battery of industrial chillers. A second apparatus was mounted to the microtome to support a digital camera and lighting system directly above the microtome stage; it was designed to acquire high-resolution images of the surface of the block (gelatin and brain) through the entire slicing procedure. These images were the basis for 3D reconstruction and currently serve as a digital catalogue representing the collection of tissue slices. Image acquisition and volume reconstruction Tomographic images were acquired using a digital single-lens reflex camera (Nikon D700, Nikon Inc., Melville, NY) bearing a 35-mm lens (AF NIKKOR 35 mm f/2D), which was connected to a PC workstation and controlled remotely. A pair of opposite, light-emitting diode arrays were pointed at the surface of the block at an angle of 45°, providing constant illumination during the cutting procedure. The image acquisition sequence was fully automated; exposure was triggered before each new stroke was initiated. Image files were saved directly on disk in raw (uncompressed) format measuring 4,256 × 2,832 pixels (equivalent to a resolution of 46 μm per pixel). The microtome camera assembly was designed to trigger each exposure every time the microtome stage stopped at a fixed position so that the resulting image stack was registered mechanically. Dedicated team members maintained a log detailing file acquisition and inspected every newly acquired image in real time. Later, we used the quality control report to identify image artifacts in the series so that ad hoc post-processing routines for 3D reconstruction could be applied. A Canon XLH1A digital HD camcorder (Canon U.S.A., Inc. Lake Success, NY) was used to record the procedure and provide a live feed of a close up of the brain within the microtome assembly on the web. Two additional views, of the microtome console and a wide-angle view of the lab, were provided via Microsoft LifeCam Cinema webcams (Microsoft Inc. Redmond, WA). The video from each of the three views was converted to flash with Adobe Flash Media Live Encoder 3.1 and streamed using Adobe Flash Media Server 3.5 (Adobe Systems Incorporated, San Jose, CA, USA). Images acquired during the cutting procedure were transferred to a Dell PowerEdge 7500 workstation running a Windows 7, 64-bit operating system with 192 GB of DDR3 dynamic random-access memory (DRAM). The digital 3D volume representing the whole brain was assembled using AMIRA. Scaling factors were derived from the in-plane resolution of the images (converted from pixels to mm) and the slicing interval (that is, section thickness). The resolution of the data set was 46 × 46 × 70μm and occupied ∼ 56 GB on disk. Access to large amounts of DRAM allowed for the efficient manipulation and inspection of the entire anatomical volume. Measurements were conducted on a volume created from images that were down-sampled to 2,550 × 2,550 pixels (voxel dimensions were x : 56.9 μm; y : 56.9 μm and z : 70 μm). The images were cropped to the edge of the gelatin block and corrected for any changes in brightness produced by fluctuations in ambient lighting that occurred during the 3-day procedure. As the ratio between brain tissue and gelatin matrix varied considerably at different levels of the series of anatomical images, we created a mask for brain tissue only and used it to adjust levels across the series. This process produced a uniform volumetric data set that was consistent in terms of luminosity and contrast in any arbitrary plane. Close inspection of the final 3D reconstruction identified occasional shifts in alignment, most likely due to accidental mechanical shifts in the equipment. Consequently, the position of outlier images was corrected by applying 2D rigid transformations (translation and rotation). The transformation matrix was computed with a local search algorithm that used a least-squares metric to compare intensities between each pair of consecutive images. 3D measurements of the hippocampus The delineation of hippocampal structures was performed on the 3D reconstruction created from the series of digital images acquired in the course of the slicing procedure. Three main orthogonal planes were visualized concurrently in the segmentation editor of AMIRA to ensure accuracy. In the coronal plane, the hippocampus was identified starting at the posterior-most level of the mammillary bodies and the structure withered at the level of the inferior colliculi. The delineation of the inferior medial border (that is, the border between the subiculum and parahippocampal cortex) was aided by the identification of the perforant pathway in the anatomical images and changes in cytoarchitecture in corresponding Nissl-stained sections. Sagittal views afforded a clear demarcation of the hippocampus’ posterior border ( Fig. 3 ); the alveus was included in the calculation of the volume [45] . The volume of the hippocampus in each hemisphere was calculated as the number of tissue voxels comprised in the delineations multiplied by the individual voxel dimensions in mm. The anatomical central axis of the hippocampus was defined as a 3D curve fit with a given stiffness along a path through the field of labelled voxels. We calculated a straight-line path using principal component analysis of a binary segmentation of the region of interest. The 3D line was sampled at uniform intervals (10 voxels) to define control points. The first and last control points of the line were set to the 3D locations defined by the furthermost extent of the object along the line. To improve the location of the control points, we sectioned the object at positions halfway between each pair of control points, using a plane that was orthogonal to the curve’s tangent direction at that location, and yielding one section for each control point. For each section of the binary object, we calculated its centre of mass and moved the corresponding control point towards that location. After the adjustments of all control points, a curve-smoothing operation was executed that used the predefined stiffness constraint on the curve. The extent of smoothing controlled the stiffness attached to the curve. The sectioning, adjustment and smoothing steps were repeated until convergence was achieved. This expectation–maximization approach iteratively adjusted the location of the curve’s control points towards a solution that intersected the object uniformly and had a given stiffness. The resulting 3D curve defined the ‘geodesic’ axis of the region of interest, and it was the basis for the actual anatomical length measurement. J.A. designed the neuroanatomical study and major instrumentation. M.P.F. conducted the brain extraction at autopsy assisted by J.A. Serial sectioning and tomographic imaging of the brain specimen was performed by J.A. with the assistance of N.M.S., P.M., N.T., J.K., A.G. and N.B., H.B., N.M.S., P.M. and J.A. developed the 3D model of the brain from cross-sectional image data acquired during the dissection. H.B. developed the 3D measurement and image registration tools. J.A., P.M. and C.S produced the stained histological slides. J.A. wrote the manuscript with significant editing contributions by S.C. and M.P.F. Photographs and figures were created by J.A. and C.S. Additional background research was conducted by R.K. How to cite this article: Annese, J. et al. Postmortem examination of patient H.M.’s brain based on histological sectioning and digital 3D reconstruction. Nat. Commun. 5:3122 doi: 10.1038/ncomms4122 (2014).